The dual role of coherent twin boundaries in hydrogen embrittlement Hydrogen embrittlement (HE) causes engineering alloys to fracture unexpectedly, often at considerable economic or environmental cost. Inaccurate predictions of component lifetimes arise from inadequate understanding of how alloy microstructure affects HE. Here we investigate hydrogen-assisted fracture of a Ni-base superalloy and identify coherent twin boundaries (CTBs) as the microstructural features most susceptible to crack initiation. This is a surprising result considering the renowned beneficial effect of CTBs on mechanical strength and corrosion resistance of many engineering alloys. Remarkably, we also find that CTBs are resistant to crack propagation, implying that hydrogen-assisted crack initiation and propagation are governed by distinct physical mechanisms in Ni-base alloys. This finding motivates a re-evaluation of current lifetime models in light of the dual role of CTBs. It also indicates new paths to designing materials with HE-resistant microstructures. Uptake of hydrogen (H) can cause engineering alloys to lose their ductility and fracture unexpectedly [1] . This deleterious phenomenon, known as hydrogen embrittlement (HE), disrupts power generation, H containment and hydrocarbon extraction [2] , [3] , [4] . High-strength alloys subjected to HE in extreme environments, such as deep oil wells, are often poorly accessible and difficult to monitor, forcing reliance on conservative lifetime limits to prevent catastrophic failures [5] , [6] . Inadequate understanding of how alloy microstructure affects HE hampers higher-fidelity component lifetime predictions. Coherent twin boundaries (CTBs) are often thought to be inherently resistant to HE because of their high surface separation energy and low H solubility [7] , [8] . However, we show that in Inconel 725—an advanced nickel (Ni)-base alloy developed specifically for extreme environments [9] —cracks preferentially initiate at Σ3 CTBs, yet at the same time are unlikely to propagate along them. By elucidating the surprising dual role of Σ3 boundaries in HE, our work demonstrates that H-assisted crack initiation and propagation are governed by distinct physical mechanisms in this alloy system. This finding opens new paths to improved failure prediction and to design of HE-resistant materials. Mechanical testing of hydrogen embrittled samples We conducted in situ tensile tests on H-charged samples of Inconel 725 in a scanning electron microscope (SEM; see Methods). The samples were prepared with different thicknesses: a thin sample (30 μm) that contains mostly through-thickness grains and a thicker sample (45 μm) where most grains do not extend through the sample thickness. No evidence of intergranular fracture was observed in samples that were not charged with H: failure in them was ductile-transgranular and occurred after onset of necking ( Supplementary Fig. 1 ). By contrast, H-charged samples did not neck and exhibited a mixture of ductile transgranular and brittle-like intergranular fracture, as shown in Fig. 1 . Such behaviour is common in HE of face-centred cubic (FCC) metals, such as Ni and Ni-base alloys [10] , [11] . In the thicker sample, we observed a large number of intergranular secondary cracks in addition to the main crack ( Fig. 1a ). These secondary cracks enabled us to pinpoint the microstructural features responsible for crack initiation and propagation. 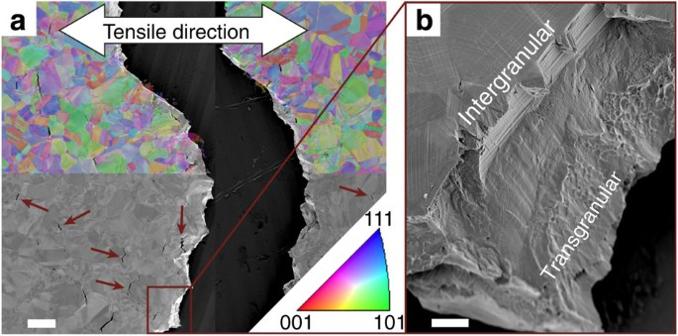Figure 1: Post-mortem EBSD analysis of H-charged Inconel 725. (a) EBSD maps superimposed on SEM micrographs from a 45-μm-thick sample loaded to failure in tension showing both the main crack and several secondary cracks (identified by arrows). The colour map indicates out-of-plane orientations of grains. Scale bar, 100 μm. (b) Higher magnification SEM image of the boxed region inaillustrating mixed intergranular and transgranular fracture along the main crack. Scale bar, 10 μm. Figure 1: Post-mortem EBSD analysis of H-charged Inconel 725. ( a ) EBSD maps superimposed on SEM micrographs from a 45-μm-thick sample loaded to failure in tension showing both the main crack and several secondary cracks (identified by arrows). The colour map indicates out-of-plane orientations of grains. Scale bar, 100 μm. ( b ) Higher magnification SEM image of the boxed region in a illustrating mixed intergranular and transgranular fracture along the main crack. Scale bar, 10 μm. Full size image Secondary crack analysis To distinguish between crack initiation and propagation sites, we classify all secondary cracks as ‘single-grain boundary (GB) cracks’ or ‘multi-GB cracks,’ based on the number of cracked GBs they contain. Single-GB cracks contain just one partially or fully cracked GB, as illustrated in Fig. 2a–c , and may terminate in a short intragranular crack. Dark regions in the electron backscatter diffraction (EBSD) map represent areas with insufficient signal to determine grain orientation, due either to lack of material in the case of cracks or to surface contamination resulting from sample handling. As there are no pre-existing cracks in our samples and H-assisted cracks initiate at the sample surface [12] , the GBs in the single-GB cracks are identified as preferential crack initiation sites. We consider crack initiation to encompass the nucleation and initial growth of a crack along a single GB, and initiation sites to be the microstructural features at which this occurs. We do not find any intergranular crack initiation at or propagation through brittle μm-scale carbides ( Supplementary Fig. 2 ), in contrast to previous observations in steel [13] , nor do we find cracks initiating along slip bands, as observed in iron-based superalloys [14] . After initiation, intergranular cracks may propagate along adjacent GBs and thus become multi-GB cracks, as shown in Fig. 2d–f . From these cracks, we determine which GBs are especially susceptible to crack propagation. Finally, we also investigate the character of non-cracked GBs connected to the ends of single- and multi-GB cracks. These GBs are likely to be crack propagation resistant, as cracks adjacent to them did not propagate along them. 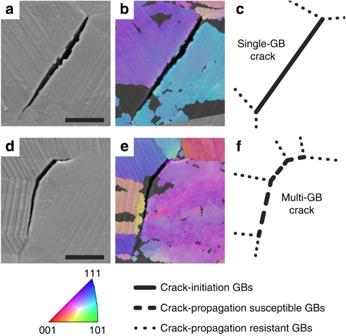Figure 2: Two categories of secondary cracks. SEM and EBSD analysis of a representative (a–c) single-GB and (d–f) multi-GB crack. (a,d) SEM micrographs with (b,e) overlaid EBSD maps are used to identify cracked and connected, non-cracked, GBs in secondary cracks. (c,f) Corresponding schematic representations. Scale bars, 5 μm. Figure 2: Two categories of secondary cracks. SEM and EBSD analysis of a representative ( a – c ) single-GB and ( d – f ) multi-GB crack. ( a , d ) SEM micrographs with ( b , e ) overlaid EBSD maps are used to identify cracked and connected, non-cracked, GBs in secondary cracks. ( c , f ) Corresponding schematic representations. Scale bars, 5 μm. Full size image H-assisted fracture susceptibility of different GB types We characterized all GBs of interest, cracked and non-cracked, by correlating SEM images with EBSD data (see Methods). GBs were classified based on their Σ value, which is a measure of misorientation in coincidence site lattice theory [15] . GBs with Σ=1–29 are labelled as ‘low-Σ’ and all others as ‘general.’ Among low-Σ GBs, we call particular attention to Σ3 CTBs because they are often thought to improve mechanical strength and resistance to stress corrosion cracking in metal alloys [16] . These qualities stem from the especially low energy of Σ3 CTBs, which is due to perfect, atom-to-atom registry between adjoining crystals at such boundaries [17] . As shown in Fig. 3a , a surprisingly large fraction—19 out of 33, that is, ~58%—of single-GB cracks are along low-Σ GBs. Moreover, 13 (~40%) of them lie along Σ3 CTBs, suggesting that CTBs are preferential crack initiation sites. To assess the statistical significance of this conclusion, we compare the fraction of Σ3 CTBs in single-GB cracks with their fraction in the microstructure as a whole ( Supplementary Note 1 ). Had cracks initiated at any GB in the microstructure with equal likelihood, then the probability or ‘ P -value’ of finding 13 Σ3 CTBs at 33 single-GBs cracks would be <0.05 ( Supplementary Table 1 ). Thus, we conclude that Σ3 CTBs are indeed preferential crack initiation sites. 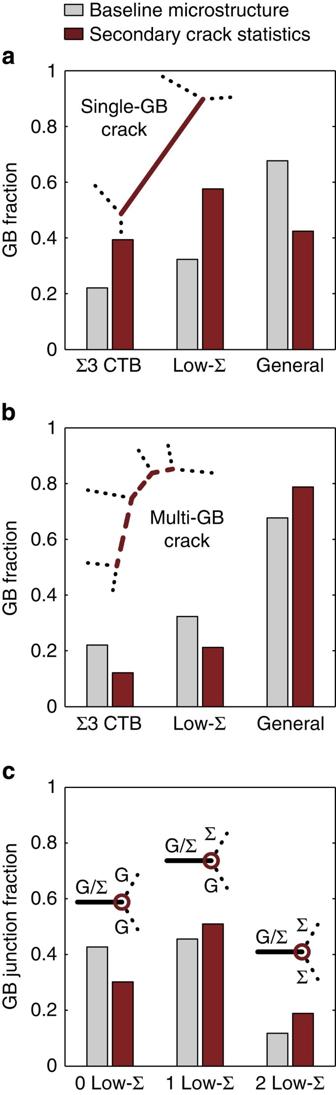Figure 3: Statistical analysis of crack initiation and propagation. Fraction of GB types that (a) initiate cracks or (b) are susceptible to crack propagation (red bars) compared with their occurrence in the baseline microstructure (grey bars). (c) Fraction of three different types of GB junctions at crack termination nodes (red bars) according to the number of low-Σ (‘Σ’) as opposed to general (‘G’) GBs that they contain compared with their occurrence in the baseline microstructure (grey bars). Figure 3: Statistical analysis of crack initiation and propagation. Fraction of GB types that ( a ) initiate cracks or ( b ) are susceptible to crack propagation (red bars) compared with their occurrence in the baseline microstructure (grey bars). ( c ) Fraction of three different types of GB junctions at crack termination nodes (red bars) according to the number of low-Σ (‘Σ’) as opposed to general (‘G’) GBs that they contain compared with their occurrence in the baseline microstructure (grey bars). Full size image To unambiguously identify the initiation site of the primary crack, we performed an in situ tensile test on a thin (30 μm) sample with through-thickness grains. All the GBs are visible on the surface of this sample and no secondary cracks are observed. The main crack initiates along a Σ3 and a Σ9 boundary, in agreement with the results reported in Fig. 3 , and then quickly propagates across the sample ( Supplementary Movie 1 and Supplementary Fig. 3 ). To determine GB susceptibility to crack propagation, we analysed multi-GB cracks using a similar procedure to that used for crack initiation. If a specific GB type is crack-propagation resistant, we expect it to occur less frequently in multi-GB cracks than in the microstructure as a whole. Figure 3b shows that 52 out of 66 (~79%) cracked GBs in multi-GB cracks are general GBs, whereas only 14 (~21%) are low-Σ and 8 (~12%) are Σ3 CTBs. The P -values corresponding to these results are as low as ~0.03 ( Supplementary Table 2 ), demonstrating quantitatively that the likelihood of crack propagation along low-Σ and Σ3 CTBs is indeed lower than for general GBs. Interestingly, the incidence of low-Σ GBs in multi-GB cracks is consistent with the frequency of crack initiation at low-Σ GBs, suggesting that when low-Σ GBs do appear in multi-GB cracks, it is likely that they are the initiation sites. Indeed, only 3 out of 66 multi-GB cracks contain more than one low-Σ GB. We also analyse the GB junctions at the tips of secondary cracks (both in single- and multi-GB cracks) to assess the role of GB connectivity in crack propagation. We categorize these junctions according to the number of low-Σ boundaries among the boundaries ahead of the crack tip: zero, one or two. Figure 3c compares the types of GB junctions found at the crack tips of all 99 secondary cracks from the thicker sample with their expected occurrence in the microstructure as a whole ( Supplementary Note 2 ). GB junctions with two low-Σ boundaries at the crack tip occur more frequently than such junctions occur in the microstructure ( P -value=0.09; Supplementary Table 3 ). Conversely, GB junctions with no low-Σ boundaries occur less frequently at crack tips than they occur in the microstructure ( P -value=0.04; Supplementary Table 3 ). This observation is consistent with low-Σ GBs being crack propagation resistant, and supports the notion that GB connectivity is an important factor affecting crack propagation in HE. Previous work on pure Ni showed that increasing the fraction of low-Σ boundaries reduces HE susceptibility [18] . Our study reveals a more subtle relationship between microstructure and HE: low-Σ boundaries and, most surprisingly Σ3 CTBs, play a dual role in H-assisted fracture. In Inconel 725, they are weak against crack initiation and strong against crack propagation. A dramatic illustration of this duality may be seen in Fig. 4 , where two distinct cracks initiate along one especially long Σ3 CTB, yet neither crack propagates far enough to fracture the GB completely. Instead, they both terminate in short intragranular cracks. 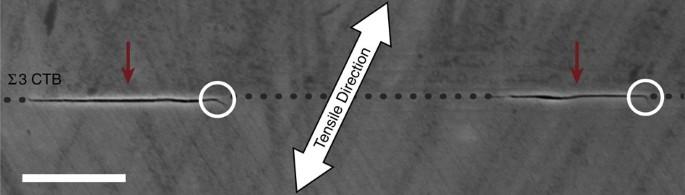Figure 4: The dual role of Σ3 CTBs in H-charged Inconel 725. SEM micrograph illustrating the duality of Σ3 CTBs in crack initiation and propagation: two single-GB cracks (identified by red arrows) initiate along one long Σ3 CTB (dotted line). However, neither crack propagates along the entire Σ3 CTB. Instead, both cracks terminate in short intragranular segments (white circles). Scale bar, 10 μm. Figure 4: The dual role of Σ3 CTBs in H-charged Inconel 725. SEM micrograph illustrating the duality of Σ3 CTBs in crack initiation and propagation: two single-GB cracks (identified by red arrows) initiate along one long Σ3 CTB (dotted line). However, neither crack propagates along the entire Σ3 CTB. Instead, both cracks terminate in short intragranular segments (white circles). Scale bar, 10 μm. Full size image The greater resistance of low-Σ GBs—and particularly Σ3 CTBs—to crack propagation, as compared with general GBs, may be due to their higher surface separation energies [7] and lower H solubility [8] . However, the same properties might be expected to make Σ3 boundaries resistant to crack initiation, contrary to our findings. The fact that a single GB type may at the same time be a preferential crack initiation site and a poor propagation path implies that the mechanisms governing crack initiation and propagation in H-charged Inconel 725 are fundamentally different. The mechanism by which H preferentially causes crack initiation at Σ3 CTBs has yet to be fully understood. An analogy may be made to fatigue in FCC-base alloys, where Σ3 CTBs are also found to initiate cracks [19] , [20] . Under cyclic loading, crack initiation at CTBs has been tied to localization of dislocation activity along persistent slip bands that intersect CTBs and within the boundaries themselves [21] , [22] , [23] . The striking similarity in the behaviour of Σ3 CTBs under fatigue and HE suggests that hydrogen induces plastic flow localization comparable to that in fatigue, even in the case of monotonic loading [24] . Indeed, hydrogen is well known to enhance dislocation activity [25] , [26] and to give rise to much higher dislocation densities than would be expected based on the uniform plastic strain applied [27] . To shed additional light on the role of plasticity in crack initiation, we measured the inclination angle of single-GB cracks relative to the tensile direction in our experiments. The results, shown in Fig. 5 , indicate that cracks initiating on CTBs are often inclined at ~60° to the tensile axis. Therefore, under uniaxial tension, these GBs experience significant shear tractions, in addition to normal tractions. Shear loading may cause the two crystal grains that meet at the boundary to slide past each other. In the case of CTBs, such sliding may occur by dislocation glide along the GB plane, that is, by the conventional dislocation-based mechanism of plastic deformation [28] , [29] , [30] , [31] . Dislocation-mediated GB sliding is possible at CTBs because the GB plane of a CTB is a {111} plane, that is, a glide plane for dislocations in FCC metals [32] . 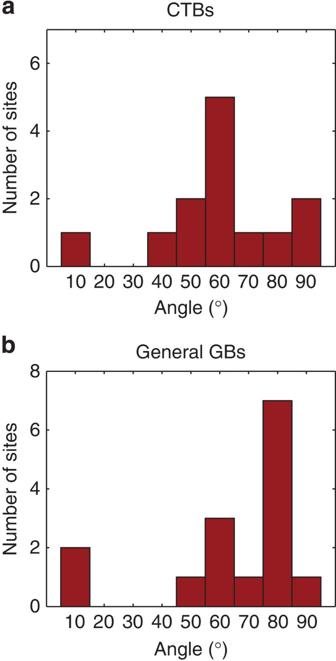Figure 5: The role of plasticity in crack initiation. Inclination angle with respect to the tensile axis of single-GB cracks on (a) CTBs and (b) general GBs. Figure 5: The role of plasticity in crack initiation. Inclination angle with respect to the tensile axis of single-GB cracks on ( a ) CTBs and ( b ) general GBs. Full size image Enhanced dislocation activity along CTBs may promote intergranular fracture in several ways. For example, the accumulation of extrinsic dislocations increases the local hydrogen concentration and alters GB structure, elevating GB energy [27] , [33] , [34] , [35] , [36] . Both of these factors are expected to decrease GB cohesive energy and promote decohesion. The fact that crack initiation occurs mostly at CTBs oriented at oblique angles with respect to the tensile axis, as seen in Fig. 5 , shows that some slip along the boundary is necessary before conditions favouring decohesion are established. Another plasticity mechanism that may play a role in crack initiation is slip transmission and plastic flow localization. Previous studies have pointed to the importance of the orientation of slip systems relative to the GB plane in controlling susceptibility to integranular cracking [37] , [38] , [39] . In these studies, favourably oriented slip channels impinging on GBs cause incorporation of dislocations directly into the boundary plane. CTBs transmit dislocations on some slip systems easily, but constitute strong barriers to dislocation motion on others [29] . Dislocations that are not transmitted may remain trapped at the CTB plane. Because CTB planes are dislocation glide planes in Inconel 725, we expect that trapped dislocations are able to glide more easily within CTBs than dislocations trapped in general GBs. The high mobility of trapped dislocations at CTBs may promote the formation of dislocation substructures in the boundary plane, similar to those formed by cyclic loading within persistent slip bands [21] . It has been suggested that γ ′ precipitates, which are present in Inconel 725 (ref. 40 ), may also play a role in crack initiation on Σ3 CTBs [41] . The effect of dislocation plasticity on crack initiation may be far more complex when multiple cracks initiate along the same GB, as shown in Fig. 4 . In such cases, different levels of crack tip shielding than at isolated cracks may be expected due to the interaction of dislocation densities surrounding neighbouring cracks [42] , [43] , [44] . This interaction may include—among other possibilities—enhanced annihilation of opposite sign dislocations [45] , generation of a greater number of statistically stored ‘redundant’ dislocations [46] , repulsion of like-signed dislocations and modified levels of cross-slip. In contrast to CTBs, Fig. 5 shows that general GBs are more often found to be nearly normal to the tensile axis. Thus, failure at such boundaries is promoted predominantly by tension, rather than shearing, and classical H-induced decohesion (that is, without the influence of slip along the boundary plane) may play a more significant role in fracture. This view is consistent with the fact that slip along general GBs is typically more complex than in CTBs and may involve dislocation climb or localized shear transformations, both of which are expected to be more difficult than dislocation glide. Moreover, in contrast to CTBs, stress concentrations formed by impinging dislocations may be accommodated more easily by the more disordered atomic structure of general GBs, averting crack initiation [47] , [48] . The identification of preferential crack initiation and propagation sites in Inconel 725 has far-reaching technological implications. Nickel-base superalloys are among the most HE-resistant structural materials in use today [9] and elucidating the dual role of CTBs in HE will enable higher accuracy lifetime predictions for these materials. Our findings also indicate new paths to improving HE-resistance through microstructure design. H-induced cracks often initiate at surfaces and propagate inward [12] . Thus, microstructurally graded materials with few Σ3 CTBs at surfaces and a large number in the interior may be less susceptible to H-assisted fracture. Tailored densities and distributions of Σ3 CTBs may be achieved through specialized thermomechanical treatments [49] . Other approaches would optimize not only the number of Σ3 CTBs, but also their connectivity [50] , with the goal of maximizing the number of GB junctions that arrest cracks while keeping the total number of Σ3 CTBs to a minimum to reduce crack initiation. Our study also motivates a closer examination of the role GB character plays in HE in Ni-base alloys and pinpoints CTBs as key microstructural features governing HE to be studied in further detail. Sample preparation and characterization Inconel 725 samples were obtained from Special Metals Corporation. Three dogbone-shaped specimens with a gage length of 15 mm and width of 1.7 mm were cut out using electrical discharge machining. They were mechanically ground to 30 and 45 μm thickness and polished on both sides to 0.04 μm with a colloidal silica suspension. After polishing, two samples were cathodically charged with hydrogen (H) for 12 h at a current density of 100 mA cm −2 in 1 N H 2 SO 4 . The third sample was tested with no hydrogen. Under these conditions, the H-charging depth is expected to be on the order of ~10 μm. These charging conditions were chosen based on a HE study in a closely related alloy [12] , which reported comparable mechanical behaviour ( Supplementary Fig. 4 ). Before testing, the sample microstructure was characterized by EBSD using a step size of 2 μm with a Philips XL30 SEM. The GB network and GB character distribution were analysed using MTex 3.4.1 in Matlab 2013b. GBs were classified according to the coincident site lattice theory using Brandon’s criterion, which sets the angular tolerance for a Σ n boundary equal to (refs 51 , 52 ). EBSD allowed to characterize all GBs at the sample surface on large areas (~1.7 × 1.9 mm 2 ). EBSD characterization was performed both before H charging and mechanical testing as well as after the samples were tested to failure. This allowed precise correlation of the location of primary and secondary cracks with the GB network. In some cases, high-magnification scans were also acquired to resolve small secondary cracks that were not visible from large-area scans. The chemical composition of several representative GBs (a Σ3 CTB, a Σ27 and four general GBs) was analysed using Electron Dispersive Spectroscopy and Electron Energy Loss Spectroscopy in a Transmission Electron Microscope. These investigations showed no detectable segregation of impurities at any of the analysed boundaries. Mechanical testing In situ tensile tests were performed using a Gatan Microtest 300 tensile testing module in a JEOL 6610LV SEM. The samples were strained at a rate of ~1 × 10 −4 s −1 . This same testing condition was used in another HE study in a closely related alloy [12] . When no H was introduced, the sample failed at approximately 4.25% total engineering strain. H-charged samples failed at approximately 1.85% and 2.6% total engineering strain, for samples with thickness 30 and 45 μm, respectively. Stress–strain curves are presented in Supplementary Fig. 4 . The sample with no H did not show any evidence of intergranular fracture and failed by ductile, transgranular fracture after onset of necking ( Supplementary Fig. 1 ). No secondary cracks were found in the sample with no H. The thicker H-charged sample (45 μm thick) exhibited more plastic deformation before failure, resulting in the formation of a large number of secondary cracks around the main crack ( Fig. 1 ). These samples were therefore used for the statistical study of secondary cracks. The thinner H-charged sample (30 μm thick) was used to identify the initiation site of the main crack. This is evidenced in Supplementary Fig. 3 , where the primary crack initiation site was identified through inspection of the in situ straining video ( Supplementary Movie 1 ) and the post-mortem characterization of the fracture surface. How to cite this article: Seita, M. et al . The dual role of coherent twin boundaries in hydrogen embrittlement. Nat. Commun. 6:6164 doi: 10.1038/ncomms7164 (2015).